Nuclear factor Y-mediated H3K27me3 demethylation of theSOC1locus orchestrates flowering responses ofArabidopsis Nuclear factor Y (NF-Y) is a conserved heterotrimeric transcription factor complex that binds to the CCAAT motifs within the promoter region of many genes. In plants, a large number of genes code for variants of each NF-YA, B or C subunit that can assemble in a combinatorial fashion. Here, we report the discovery of an Arabidopsis NF-Y complex that exerts epigenetic control over flowering time by integrating environmental and developmental signals. We show that NF-Y interacts with CONSTANS in the photoperiod pathway and DELLAs in the gibberellin pathway, to directly regulate the transcription of SOC1 , a major floral pathway integrator. This NF-Y complex binds to a unique cis -element within the SOC1 promoter to modulate trimethylated H3K27 levels, partly through a H3K27 demethylase REF6. Our findings establish NF-Y complexes as critical mediators of epigenetic marks that regulate the response to environmental or intrinsic signals in plants. The transition from vegetative to reproductive development is crucial for reproductive success of flowering plants. In Arabidopsis , the timing of this transition is controlled by a complex network of flowering genetic pathways in response to developmental cues and environmental signals [1] . The interactions among these flowering pathways regulate the expression of two floral pathway integrators, FLOWERING LOCUS T ( FT ) and SUPPRESOR OF OVEREXPRESSION OF CONSTANS 1 ( SOC1 ), which in turn activate the genes involved in the formation of floral meristems [2] , [3] , [4] , [5] . The major flowering pathways include photoperiod and gibberellin (GA) pathways that promote flowering in response to seasonal changes in day length and the endogenous phytohormone GA, respectively. CONSTANS (CO) plays a central role in mediating photoperiod-dependent flowering [6] . When CO messenger RNA (mRNA) expression regulated by the circadian clock coincides with the exposure of plants to light under long days (LDs), the CO protein is stabilized in the nucleus and upregulates downstream genes, including FT and SOC1 , to promote flowering [3] , [7] , [8] . Both CO in the photoperiod pathway and PHYTOCHROME INTERACTING FACTOR4 in the thermosensory pathway directly activate the mRNA expression of FT that encodes the protein as part of the florigen in leaves [3] , [9] , [10] , [11] . Long-distance movement of FT protein from leaves to the shoot apex through the phloem system allows FT to interact with a bZIP transcription factor FD in the shoot apical meristem for activating floral meristem identity genes [10] , [12] , [13] . SOC1 is expressed in leaves and shoot apical meristems in response to multiple flowering pathways, and encodes a MADS-box transcription factor that acts as a key flowering promoter through regulating another floral meristem identity gene, LEAFY [2] , [3] , [4] , [5] , [14] , [15] , [16] . Although several studies indicate that CO activates SOC1 either directly or indirectly via FT in the photoperiod pathway [3] , [10] , [17] , [18] , so far there is no evidence to support direct regulation of SOC1 transcription by CO or FT. The GA pathway also plays an important role in the promotion of flowering in Arabidopsis under both LDs and short days, although its effect under LDs is usually masked by the photoperiod pathway [19] , [20] . Molecular genetic analyses of GA and photoperiod pathways suggest that the photoperiod and GA pathways are coordinated to promote flowering under LDs [15] , [20] , [21] . The GA effect on flowering is genetically mediated by five DELLA proteins, GIBBERELLIC ACID INSENSITIVE (GAI), REPRESSOR OF ga1-3 (RGA), RGA-LIKE1 (RGL1), RGL2 and RGL3, which are key GA signalling repressors whose degradation is triggered by GA [22] , [23] . As transcriptional regulators, DELLA proteins have been shown to exert their function by recruiting other transcription factors rather than directly binding to their target genes [24] , [25] , [26] , [27] . It has been suggested that photoperiod-dependent flowering involves nuclear factor Y (NF-Y) complexes, which are conserved combinatorial transcription factors in eukaryotes consisting of NF-YA, NF-YB and NF-YC subunits [28] , [29] , [30] , [31] , [32] . NF-Y and its binding element, the CCAAT box, are among the first set of trans -acting factors and cis -elements identified in eukaryotes [33] . The Arabidopsis genome contains 10 NF-YA, 13 NF-YB and 13 NF-YC subunits, which could theoretically form 1,690 unique heterotrimeric NF-Y transcription factors, potentially enabling the specific control of a variety of target genes [32] , [34] . In this study, we report the discovery of a complete NF-Y complex consisting of three different subunits that regulates flowering time in response to photoperiod and GA pathways in Arabidopsis . NF-Y subunits interact with CO and DELLAs to directly regulate SOC1 expression. The NF-Y complex binds to a unique cis -element in the SOC1 promoter through its NF-YA2 subunit, and modulates H3K27me3 dynamics at SOC1 partly via RELATIVE OF EARLY FLOWERING 6 (REF6), a H3K27 demethylase. Our findings uncover that the combinatorial NF-Y transcription factor plays a critical role in mediating epigenetic control of the floral transition through its interaction with key regulators in the photoperiod and GA pathways, thus orchestrating plant responses to environmental and intrinsic flowering signals. DELLAs and CO interact with NF-Y subunits DELLA proteins function as key transcriptional regulators that mediate GA effect on plant development. To further investigate the function of DELLA proteins, we performed a yeast two-hybrid screening to identify RGA-interacting partners using an inflorescence cDNA library (CD4-30 from ABRC) [26] , and found that RGA interacted with NF-YC3 and its closest homologue NF-YC9, two Arabidopsis NF-YC family members [32] , [34] , in yeast. This result, together with a recent finding describing the involvement of NF-YC3 and NF-YC9 in CO-mediated control of flowering [28] , prompted us to investigate whether DELLAs and CO coordinately interact with NF-Y subunits to regulate flowering time. To systematically study the protein interactions of representative NF-Y subunits with RGA and CO, we selected two NF-YA (A1 and A2), three NF-YB (B1, B2 and B3), and three NF-YC (C1, C3 and C9) homologues because they are either relevant with flowering time control or expressed in the vasculature similarly to CO [28] , [29] , [30] , [31] , [34] . Yeast two-hybrid assays revealed that in addition to NF-YC3 and NF-YC9 found in initial yeast two-hybrid screening, RGA also interacted strongly with NF-YA1 and NF-YA2, and weakly with NF-YB2 ( Fig. 1a ). CO not only interacted with all NF-YC subunits examined, but also interacted weakly with NF-YB2 ( Fig. 1a ). Glutathione S-transferase (GST) pull-down assays verified the protein interactions of the selected NF-YB and NF-YC subunits (NF-YB2 and NF-YC9) with RGA and CO, but did not show the interaction between RGA and the selected NF-YA subunit (NF-YA2) ( Fig. 1b ) as revealed by yeast two-hybrid assays. We further performed bimolecular fluorescence complementation (BiFC) analyses, and found the interactions of all selected NF-Y subunits (NF-YA2, NF-YB2 and NF-YC9) with RGA and CO in the nuclei of tobacco cells ( Fig. 1c , Supplementary Fig. 1 ). Therefore, these results consistently demonstrate that RGA and CO interact with NF-YB and NF-YC subunits, while the interaction of NF-YA subunits with RGA and CO may depend on other endogenous factors in plants, such as NF-YC subunits, as discussed later. 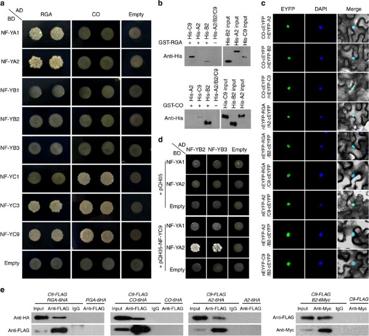Figure 1: CO and RGA interact with NF-Y subunitsin vitroandin vivo. (a) Yeast two-hybrid assays show the interactions of NF-Y subunits with RGA and CO. Transformed yeast cells were grown on SD-Trp/-Leu/-His/-Ade medium. (b)In vitropull-down assays show the interactions of NF-Y subunits with RGA and CO. His-tagged proteins were incubated with immobilized GST (−) or GST-tagged proteins (+) and immunoprecipitated fractions were detected by anti-His antibody. (c) BiFC analysis of the interactions among NF-Y subunits and between NF-Y subunits and CO or RGA in tobacco epidermal cells. Enhanced yellow fluorescence protein (EYFP), fluorescence of enhanced yellow fluorescent protein; DAPI, fluorescence of 4′,6-diamino-2-phenylindol; Merge, merge of EYFP, DAPI and bright field. (d) Yeast three-hybrid assays show the interactions between NF-YA and NF-YB subunits in the presence of NF-YC9. The empty vector pQH05 was co-transformed with AD and BD plasmids to serve as a control in the upper panel. Transformed yeast cells were grown on SD-Trp/-Leu/-His/-Ade medium. (e)In vivointeraction among NF-Y subunits and between NF-YC9 and CO or RGA inArabidopsis. Plant nuclear extracts from various 9-day-old transgenic seedlings grown under LDs were immunoprecipitated by anti-Myc antibody, anti-FLAG antibody or preimmune serum (IgG) as indicated above each blot. The co-immunoprecipitated proteins were detected by anti-FLAG, anti-Myc or anti-HA antibody as indicated on the left of the blots.C9-FLAG,nf-yc9-1 pNF-YC9:NF-YC9-FLAG; RGA-6HA,ga1-3 35S:RGA-6HA;CO-6HA,SUC2:CO-6HA;A2-6HA,35S:NF-YA2-6HA;B2-6Myc,pNF-YB2:NF-YB2-6Myc. Figure 1: CO and RGA interact with NF-Y subunits in vitro and in vivo . ( a ) Yeast two-hybrid assays show the interactions of NF-Y subunits with RGA and CO. Transformed yeast cells were grown on SD-Trp/-Leu/-His/-Ade medium. ( b ) In vitro pull-down assays show the interactions of NF-Y subunits with RGA and CO. His-tagged proteins were incubated with immobilized GST (−) or GST-tagged proteins (+) and immunoprecipitated fractions were detected by anti-His antibody. ( c ) BiFC analysis of the interactions among NF-Y subunits and between NF-Y subunits and CO or RGA in tobacco epidermal cells. Enhanced yellow fluorescence protein (EYFP), fluorescence of enhanced yellow fluorescent protein; DAPI, fluorescence of 4′,6-diamino-2-phenylindol; Merge, merge of EYFP, DAPI and bright field. ( d ) Yeast three-hybrid assays show the interactions between NF-YA and NF-YB subunits in the presence of NF-YC9. The empty vector pQH05 was co-transformed with AD and BD plasmids to serve as a control in the upper panel. Transformed yeast cells were grown on SD-Trp/-Leu/-His/-Ade medium. ( e ) In vivo interaction among NF-Y subunits and between NF-YC9 and CO or RGA in Arabidopsis . Plant nuclear extracts from various 9-day-old transgenic seedlings grown under LDs were immunoprecipitated by anti-Myc antibody, anti-FLAG antibody or preimmune serum (IgG) as indicated above each blot. The co-immunoprecipitated proteins were detected by anti-FLAG, anti-Myc or anti-HA antibody as indicated on the left of the blots. C9-FLAG , nf-yc9-1 pNF-YC9:NF-YC9-FLAG; RGA-6HA , ga1-3 35S:RGA-6HA ; CO-6HA , SUC2:CO-6HA ; A2-6HA , 35S:NF-YA2-6HA ; B2-6Myc , pNF-YB2:NF-YB2-6Myc. Full size image To test whether the selected NF-Y subunits that interact with RGA and CO could form heterotrimeric NF-Y transcription factors, we performed yeast two-hybrid assays to examine the interactions among these NF-Y subunits. NF-YC3 and NF-YC9 interacted with both NF-YA and NF-YB subunits ( Supplementary Fig. 2 ), whereas no interactions between NF-YA and NF-YB subunits were observed ( Fig. 1d , upper panel). Yeast three-hybrid assays further showed that NF-YC9 was required for the interactions between NF-YA and NF-YB subunits ( Fig. 1d ). BiFC analysis confirmed the interactions of NF-YC9 with NF-YA2 and NF-YB2 in the nuclei of tobacco cells ( Fig. 1c ). These results, together with a recent study on the bilateral interactions between NF-Y subunits [35] , suggest that NF-YC subunits directly interact with NF-YA and NF-YB subunits, and might be necessary for the interaction between NF-YA and NF-YB subunits for the assembly of the trimeric NF-Y complex. As NF-YC9 interacted with other NF-Y subunits, RGA and CO in yeast and tobacco cells ( Fig. 1a,c , Supplementary Fig. 2 ), we created pNF-YC9:NF-YC9-FLAG plants to examine the interaction of NF–YC9 with other proteins in Arabidopsis . pNF-YC9:NF-YC9-FLAG rescued the late-flowering phenotype of nf-yc3-2 nf-yc4-1 nf-yc9-1 (ref. 28 ) ( Table 1 ), indicating that NF-YC9-FLAG retains the biological function of NF-YC9. The nf-yc9-1 pNF-YC9:NF-YC9-FLAG line was crossed with various plants containing other tagged transgenes and the resulting homozygous progenies were used for co-immunoprecipitation analyses. Our results revealed the in vivo interaction of NF-YC9 with RGA, CO, NF-YA2 and NF-YB2 ( Fig. 1e , Supplementary Fig. 3 ). Taken together, these data suggest that RGA and CO interact with NF-Y subunits, and that NF-YC9 is a common partner interacting with other proteins involved. Similar to RGA, other DELLA proteins, such as GAI, RGL1 and RGL2, also interacted with NF-Y subunits ( Supplementary Fig. 4 ), implying widespread interactions between DELLAs and NF-Y. Table 1 Flowering time of various plants in this study. Full size table Interactions among CO, GA signalling and NF-Y Because previous studies have shown that CO, GA signalling, and individual NF-YB/C subunits are all involved in the control of flowering time under LDs [20] , [21] , [28] , [29] , [30] , [31] , we proceeded to study how their interactions affect flowering. We first crossed nf-ya2-1 and nf-yc9-1 (ref. 28 ) with nf-yb2-1 nf-yb3-1 that showed late flowering [30] . The resulting quadruple mutant nf-ya2-1 nf-yb2-1 nf-yb3-1 nf-yc9-1 exhibited even later flowering ( Table 1 ), indicating that the heterotrimeric complex of the NF-Y transcription factor comprising YA, YB and YC subunits play an important role in determining flowering time. As NF-Y subunits interacted in vivo with RGA and CO ( Fig. 1 ), we hypothesized that they could coordinately regulate certain common targets in both photoperiod and GA pathways. Thus, we tested the temporal expression of SOC1 and FT , both of which act downstream of photoperiod and GA pathways. Both SOC1 and FT were consistently downregulated in co-1 , the GA-deficient mutant ga1 , nf-yb2-1 nf-yb3-1 , and nf-ya2-1 nf-yb2-1 nf-yb3-1 nf-yc9-1 during the floral transition, whereas there was no consistent change in CO expression in these mutants ( Fig. 2a ). Furthermore, induced CO activity upregulated SOC1 and FT in a steroid-inducible co-2 35S:CO-GR line as previously reported [3] ( Fig. 2b , Supplementary Fig. 5 ). Similarly, induced RGA activity downregulated SOC1 and FT in a steroid-inducible 35S:RGA-GR line [36] in the background of ga1-3 gai-t6 rga-t2 ( Fig. 2b , Supplementary Fig. 5 ), in which null mutants of RGA and GAI, two major DELLA proteins mediating GA effect on flowering, suppressed the non-flowering defect of ga1-3 (ref. 22 ). These results demonstrate that CO, GA signalling and NF-Y all affect SOC1 and FT expression under LDs. 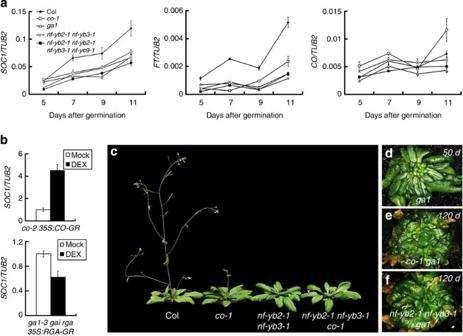Figure 2: CO, GA signalling and NF-Y regulate flowering. (a) Quantitative RT–PCR analysis of temporal expression ofSOC1,FTandCOin developing seedlings with various genetic backgrounds under LDs. The β-tubulin gene (TUB2) was amplified as an internal control. Values are mean±s.d. of three biological replicates. (b)SOC1expression inco-2 35S:CO-GRandga1-3 gai-t6 rga-t2 35S:RGA-GRseedlings. Seven-day-old seedlings grown under LDs were either mock treated or treated with 10 μM dexamethasone (DEX) for 4 h.SOC1expression was calculated by comparing the value of DEX treatment to that of mock treatment. Values are mean±s.d. of three biological replicates. (c)nf-yb2-1 nf-yb3-1 co-1exhibits comparable flowering time tonf-yb2-1 nf-yb3-1. Flowering phenotypes of representative 32-day-old plants with various genetic backgrounds grown under LDs were compared. (d–f)co-1 ga1andnf-yb2-1nf-yb3-1 ga1hardly flower as compared withga1. Flowering phenotypes of 50-day-oldga1(d), 120-day-oldco-1 ga1(e) and 120-day-oldnf-yb2-1 nf-yb3-1 ga1(f) grown under LDs were compared. Note that 50-day-oldga1has generated floral buds (d), whereasco-1 ga1(e) andnf-yb2-1 nf-yb3-1 ga1(f) do not flower within our experimental period. Figure 2: CO, GA signalling and NF-Y regulate flowering. ( a ) Quantitative RT–PCR analysis of temporal expression of SOC1 , FT and CO in developing seedlings with various genetic backgrounds under LDs. The β-tubulin gene ( TUB2 ) was amplified as an internal control. Values are mean±s.d. of three biological replicates. ( b ) SOC1 expression in co-2 35S:CO-GR and ga1-3 gai-t6 rga-t2 35S:RGA-GR seedlings. Seven-day-old seedlings grown under LDs were either mock treated or treated with 10 μM dexamethasone (DEX) for 4 h. SOC1 expression was calculated by comparing the value of DEX treatment to that of mock treatment. Values are mean±s.d. of three biological replicates. ( c ) nf-yb2-1 nf-yb3-1 co-1 exhibits comparable flowering time to nf-yb2-1 nf-yb3-1 . Flowering phenotypes of representative 32-day-old plants with various genetic backgrounds grown under LDs were compared. ( d – f ) co-1 ga1 and nf-yb2-1nf-yb3-1 ga1 hardly flower as compared with ga1 . Flowering phenotypes of 50-day-old ga1 ( d ), 120-day-old co-1 ga1 ( e ) and 120-day-old nf-yb2-1 nf-yb3-1 ga1 ( f ) grown under LDs were compared. Note that 50-day-old ga1 has generated floral buds ( d ), whereas co-1 ga1 ( e ) and nf-yb2-1 nf-yb3-1 ga1 ( f ) do not flower within our experimental period. Full size image We then investigated genetic interactions among CO, GA signalling and NF-Y. Consistent with the role of CO in the promotion of flowering, co-1 showed late flowering, while SUC2:CO-6HA showed early flowering ( Fig. 2c , Table 1 , Supplementary Fig. 6 ). nf-yb2-1 nf-yb3-1 exhibited the comparable late-flowering phenotype to nf-yb2-1 nf-yb3-1 co-1 , and almost completely suppressed early flowering of SUC2:CO-6HA ( Fig. 2c , Supplementary Fig. 6 , Table 1 ). Consistently, upregulation of SOC1 and FT expression in SUC2:CO-6HA was greatly attenuated in a nf-yb2-1 nf-yb3-1 background ( Supplementary Fig. 6 ). These results suggest that NF-Y predominantly mediates CO effect on downstream flowering promoters. In contrast, ga1 ( Columbia (Col) background) and ga1-3 (Landsberg erecta ( L er background)), both of which exhibited late flowering to different extents, did not affect early flowering of overexpression of CO ( Fig. 2d , Table 1 ). Furthermore, both co-1 ga1 (Col background) and co-2 ga1-3 (L er background) hardly flowered under our experimental period ( Fig. 2e , Table 1 ). These results support that CO and GA signalling partially function in parallel pathways to control flowering under LDs. Since CO controlled flowering in a NF-Y-dependent manner, nf-yb2-1 nf-yb3-1 ga1 expectedly exhibited the non-flowering defect similar to co-1 ga1 under LDs ( Fig. 2f , Table 1 ). NF-Y subunits are associated with the SOC1 promoter The interaction of NF-Y subunits with RGA and CO and their effects on SOC1 and FT expression provoked us to speculate whether NF-Y serves as a convergent point to mediate flowering through regulating SOC1 and FT expression in response to both photoperiod and GA pathways. To this end, we first examined whether NF-Y subunits are directly associated with SOC1 and FT regulatory regions. Chromatin immunoprecipitation (ChIP) assays of nf-yc9-1 pNF-YC9:NF-YC9-FLAG and nf-yb2-1 pNF-YB2:NF-YB2-6Myc in which pNF-YB2:NF-YB2-6Myc rescued the late-flowering phenotype of nf-yb2-1 ( Table 1 ) revealed that both NF-YC9-FLAG and NF-YB2-6Myc were associated with the genomic region near the SOC1-5 fragment with the highest enrichment fold ( Fig. 3a ). We further created 35S:NF-YA2-6HA , 35S:NF-YC3-6HA and 35S:NF-YC9-6HA transgenic plants, all of which showed slightly early flowering and dwarf or semi-dwarf stature ( Supplementary Fig. 7 , Table 1 ), indicating that these NF-Y subunits mediate similar developmental processes. ChIP assays of these materials demonstrated that these NF-Y subunits tagged with 6HA bound to the same SOC1 genomic region as NF-YC9-FLAG and NF-YB2-6Myc ( Fig. 3a , Supplementary Fig. 8 ). These results and the observation on the interactions among these NF-Y subunits suggest that three different types of subunits form the heterotrimeric NF-Y complex that recognizes the same binding region in the SOC1 promoter. 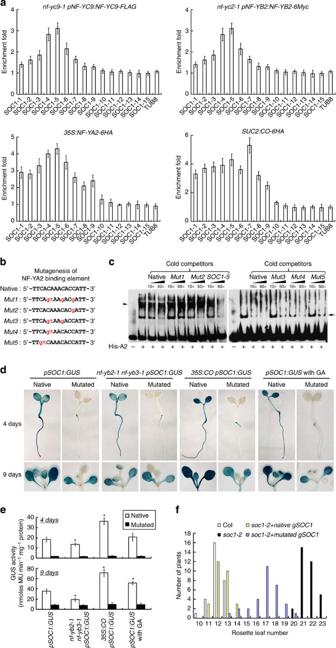Figure 3: CO and GA signalling regulateSOC1expression through NF-Y binding to theSOC1promoter. (a) ChIP analysis of binding of NF-Y subunits and CO to theSOC1regulatory regions. Nine-day-old seedlings grown under LDs were collected for ChIP analysis. Fifteen DNA fragments spanning theSOC1genomic region shown inSupplementary Fig. 8were examined by ChIP-enrichment test. Values are mean±s.d. of three biological replicates. (b) List of the putative NF-YA2 binding element (Native) inSOC1-5fragment and its mutated versions (Mut1-5) used for EMSA assays shown inc. (c) EMSA assay of the sequence elements required for NF-YA2 binding toSOC1. The biotinylated native probe was added in the absence (−) or the presence of 1 μg purified His-NF-YA2 protein (+). Various non-labelled probes (cold competitors) in 10- and 50-fold molar excess relative to the biotinylated native probe were used as competitors.SOC1-5fragment (Supplementary Fig. 11) serves as a positive control. Arrow indicates the specific binding of NF-YA2 protein to the biotinylated native probe, while arrowhead indicates non-specific bands. (d) Representative GUS staining of 4-day-old (upper panels) and 9-day-old (lower panels) seedlings containingpSOC1:GUS(Native) and its mutated construct (Mutated) in various genetic backgrounds. Seeds were germinated and grown on either MS medium or MS medium containing 10 μM GA3for the GA treatment experiment. (e) Quantitative analysis of GUS activity in variouspSOC1:GUSplants shown in (d). Values were mean±s.d. from at least 30 plants of each genotype or treatment. Asterisks indicate significant changes in GUS activity in comparison with respective controls (two-tailed Student’st-test,P<0.05). There is no statistically significant difference in GUS activity among plants containing the mutatedpSOC1:GUSconstruct in various genetic backgrounds. (f) Distribution of flowering time in T1 transgenic plants containing a 6.6-kbSOC1genomic fragment (native gSOC1) and its derived version with the mutated NFYBE (mutated gSOC1) in thesoc1-2mutant background. Figure 3: CO and GA signalling regulate SOC1 expression through NF-Y binding to the SOC1 promoter. ( a ) ChIP analysis of binding of NF-Y subunits and CO to the SOC1 regulatory regions. Nine-day-old seedlings grown under LDs were collected for ChIP analysis. Fifteen DNA fragments spanning the SOC1 genomic region shown in Supplementary Fig. 8 were examined by ChIP-enrichment test. Values are mean±s.d. of three biological replicates. ( b ) List of the putative NF-YA2 binding element ( Native ) in SOC1-5 fragment and its mutated versions ( Mut1-5 ) used for EMSA assays shown in c . ( c ) EMSA assay of the sequence elements required for NF-YA2 binding to SOC1 . The biotinylated native probe was added in the absence (−) or the presence of 1 μg purified His-NF-YA2 protein (+). Various non-labelled probes (cold competitors) in 10- and 50-fold molar excess relative to the biotinylated native probe were used as competitors. SOC1-5 fragment ( Supplementary Fig. 11 ) serves as a positive control. Arrow indicates the specific binding of NF-YA2 protein to the biotinylated native probe, while arrowhead indicates non-specific bands. ( d ) Representative GUS staining of 4-day-old (upper panels) and 9-day-old (lower panels) seedlings containing pSOC1:GUS (Native) and its mutated construct (Mutated) in various genetic backgrounds. Seeds were germinated and grown on either MS medium or MS medium containing 10 μM GA 3 for the GA treatment experiment. ( e ) Quantitative analysis of GUS activity in various pSOC1:GUS plants shown in ( d ). Values were mean±s.d. from at least 30 plants of each genotype or treatment. Asterisks indicate significant changes in GUS activity in comparison with respective controls (two-tailed Student’s t -test, P <0.05). There is no statistically significant difference in GUS activity among plants containing the mutated pSOC1:GUS construct in various genetic backgrounds. ( f ) Distribution of flowering time in T1 transgenic plants containing a 6.6-kb SOC1 genomic fragment ( native gSOC1 ) and its derived version with the mutated NFYBE ( mutated gSOC1 ) in the soc1-2 mutant background. Full size image We further tested whether CO and RGA also bind to SOC1 by ChIP analysis of SUC2:CO-6HA and ga1-3 gai-t6 rgl1-1 rgl2-1 rga-t2 35S:RGA-6HA [37] . Association of CO-6HA with SOC1 spanned a ~1.7 kb promoter region from SOC1-1 to SOC1-9 fragments with an enrichment peak at around SOC1-7 ( Fig. 3a ). In contrast, association of RGA-6HA with the SOC1 genomic region was not detectable ( Supplementary Fig. 8 ). These observations imply that CO and NF-Y co-localize at the SOC1 promoter, whereas the interaction between RGA and NF-Y could be separate from NF-Y association with the SOC1 promoter. Notably, although ChIP analysis of SUC2:CO-6HA revealed the association of CO-6HA with a 9-kb FT genomic region with an enrichment peak at the FT-14 fragment, there was no significant enrichment detectable for NF-YA2, NF-YB2, and NF-YC9 ( Supplementary Fig. 9 ). Thus, these NF-Y subunits might affect FT expression in an indirect manner. The association of CO-6HA with both SOC1 and FT genomic regions implies that CO could directly regulate both genes as previously suggested [3] , [18] . This is supported by additive effects of ft soc1 mutants on delaying flowering under LDs [17] , [38] . We also found that SOC1 was significantly upregulated in ft-10 SUC2:CO-6HA compared with ft-10 ( Supplementary Fig. 10 ). This result, together with the ChIP result showing direct binding of CO to SOC1 , suggests that CO partially activates SOC1 expression independently of FT. NF-YA2 directly binds to the NFYBE of the SOC1 promoter To identify the subunit(s) of the NF-Y complex that interacts with the SOC1-5 fragment, we performed the electrophoretic mobility shift assay (EMSA) using the biotinylated SOC1-5 fragment as a probe, and found that only NF-YA2 specifically bound to SOC1-5 ( Supplementary Figs 11 and 12 ). This is consistent with a previous study showing that only NF-YA subunits contain the essential histidine residues required for NF-Y binding to DNA [39] . We further revealed that NF-YA2 only bound to the middle subfragment of SOC1 -5 that contains a 15-bp motif flanked by a pair of inverted repeat sequences ( Supplementary Figs 11 and 13 ), which could facilitate the protein-DNA interaction [40] . We then performed EMSA using this 15-bp motif and its mutated versions as probes, and found that NF-YA2 bound to the native motif rather than the mutated version ( Mut1 ) ( Fig. 3b,c ). This motif (5′-TTCACAAACACCATT-3′) was, thus, designated as the NFYBE. NF-Y binding mediates the regulation of SOC1 by CO and GA To test in vivo whether CO and GA signalling regulate SOC1 through NF-Y binding to the NFYBE in the SOC1 promoter, we used an established pSOC1:β-glucuronidase ( GUS ) construct in which the GUS reporter gene was driven by a 2-kb SOC1 promoter upstream of the translational start site [5] . Based on this construct, we further created a mutated reporter gene cassette containing the Mut1 version of the NFYBE, 5′-TTCAgtAAgACgATT-3′ ( Fig. 3b ). Among 30 lines of transformants harbouring the mutated version, 28 lines displayed significantly reduced GUS staining at 4 and 9 days after germination compared with pSOC1:GUS plants ( Fig. 3d,e ), suggesting that the NFYBE is critical for promoting SOC1 expression during the floral transition. We then crossed the representative native and mutated pSOC1:GUS plants with nf-yb2-1 nf-yb3-1 and 35S:CO . GUS staining of pSOC1:GUS was significantly weaker in both 4- and 9-day-old nf-yb2-1 nf-yb3-1 seedlings than that in wild-type seedlings, whereas there was no significant difference in the intensity of GUS staining for the mutated pSOC1:GUS in two different genetic backgrounds ( Fig. 3d,e ). Thus, mutagenesis of the NFYBE abolishes NF-Y capacity in upregulating SOC1 , confirming that NF-Y promotes SOC1 expression through binding to the NFYBE. As expected, pSOC1:GUS displayed increased GUS staining in 35S:CO compared with wild-type seedlings, but the mutated pSOC1:GUS displayed the same weak staining in both 35S:CO and wild-type backgrounds ( Fig. 3d,e ). Furthermore, GA treatment resulted in increased GUS staining in 9-day-old pSOC1:GUS seedlings compared with non-treated seedlings, but had no effect on the mutated pSOC1:GUS seedlings. To directly test whether the NFYBE affects flowering, we transformed a 6.6-kb native SOC1 genomic fragment and its derived version with the mutated NFYBE into soc1-2 . Most of the independent soc1-2 lines transformed with the native fragment exhibited comparable flowering time as wild-type plants, whereas almost all the soc1-2 lines transformed with the mutated version flowered later than wild-type plants ( Fig. 3f ), demonstrating that mutagenesis of the NFYBE compromises the SOC1 effect on promoting flowering. Taken together, these observations strongly support that NF-Y binding to the NFYBE partly contributes to the upregulation of SOC1 in response to CO and GA signalling during the floral transition. GA signalling enhances NF-Y binding to the SOC1 promoter As our genetic analyses suggest that CO and GA signalling function in parallel pathways to control flowering under LDs ( Fig. 2e , Table 1 ), we then investigated the relative contribution of GA and CO to modulating flowering. GA treatment accelerated flowering of wild-type plants in both Col and L er backgrounds under LDs ( Supplementary Table 1 ). Consistently, GA-deficient mutants, ga1-3 (L er background) and ga1 (Col background), exhibited late flowering, while loss of function of DELLA proteins in gai-t6 rga-t2 rgl1-1 rgl2-1 exhibited early flowering ( Fig. 4a , Table 1 ). These data demonstrate that GA signalling contributes to the promotion of flowering under LDs even when the photoperiod pathway mediated by CO plays a dominant role. However, in the absence of CO, the fundamental effect of GA on flowering under LDs was clearly perceived as evident from the observations that GA treatment greatly accelerated flowering of co-1 , co-2 and co-1 ga1 ( Supplementary Table 1 ), and that gai-t6 rga-t2 rgl1-1 rgl2-1 or gai-t6 rga-t2 fully rescued the late-flowering phenotype of co-2 or the non-flowering phenotype of co-2 ga1-3 ( Fig. 4a , Table 1 ). Furthermore, SOC1 and FT expression was upregulated in gai-t6 rga-t2 rgl1-1 rgl2 regardless of CO activity ( Fig. 4b ). These observations support that GA signalling directly modulates flowering regulators, such as SOC1 , in parallel to CO. 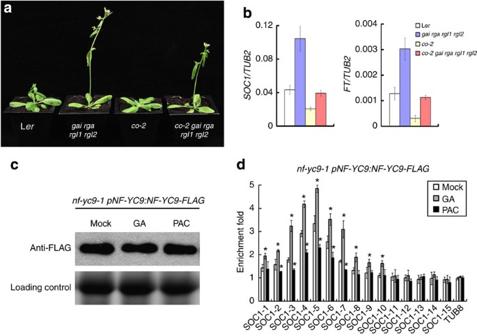Figure 4: GA signalling promotesSOC1through enhancing NF-Y binding to theSOC1promoter. (a) Loss of function of DELLAs accelerates flowering in both wild-type andco-2plants. Flowering phenotypes of representative 23-day-old plants with various genetic backgrounds grown under LDs were compared. (b) Quantitative RT–PCR analysis ofSOC1andFTexpression in 7-day-old seedlings with various genetic backgrounds under LDs.TUB2was amplified as an internal control. Values are mean±s.d. of three biological replicates. (c) Western blot analysis of NF-YC9-FLAG expression in total protein extract from 9-day-oldnf-yc9-1 pNF-YC9:NF-YC9-FLAGplants mock treated or treated with 100 μM GA3or 10 μM PAC for 24 h. (d) ChIP analysis of NF-YC9 binding to theSOC1regulatory regions innf-yc9-1 pNF-YC9:NF-YC9-FLAGplants described inc. Values are mean±s.d. of three biological replicates. Asterisks indicate significant changes in ChIP-enrichment fold in GA- or PAC-treated samples compared with mock-treated samples (two-tailed Student’st-test,P<0.05). Figure 4: GA signalling promotes SOC1 through enhancing NF-Y binding to the SOC1 promoter. ( a ) Loss of function of DELLAs accelerates flowering in both wild-type and co-2 plants. Flowering phenotypes of representative 23-day-old plants with various genetic backgrounds grown under LDs were compared. ( b ) Quantitative RT–PCR analysis of SOC1 and FT expression in 7-day-old seedlings with various genetic backgrounds under LDs. TUB2 was amplified as an internal control. Values are mean±s.d. of three biological replicates. ( c ) Western blot analysis of NF-YC9-FLAG expression in total protein extract from 9-day-old nf-yc9-1 pNF-YC9:NF-YC9-FLAG plants mock treated or treated with 100 μM GA 3 or 10 μM PAC for 24 h. ( d ) ChIP analysis of NF-YC9 binding to the SOC1 regulatory regions in nf-yc9-1 pNF-YC9:NF-YC9-FLAG plants described in c . Values are mean±s.d. of three biological replicates. Asterisks indicate significant changes in ChIP-enrichment fold in GA- or PAC-treated samples compared with mock-treated samples (two-tailed Student’s t -test, P <0.05). Full size image Although both CO and RGA interacted with NF-Y subunits ( Fig. 1 ) and regulated SOC1 expression through NF-Y binding to SOC1 ( Fig. 3b–e ), the SOC1 promoter was only associated with CO and NF-Y, but not RGA ( Fig. 3a , Supplementary Fig. 8 ). To understand how the interaction between RGA and NF-Y regulates SOC1 expression, we first examined whether treatment of GA or an inhibitor of GA biosynthesis, paclobutrazol (PAC), affects the protein levels of NF-YC9 that interacted in vivo with RGA ( Fig. 1e ). Neither GA treatment that degraded DELLA proteins including RGA nor PAC treatment that stabilized DELLA proteins affected the abundance of NF-YC9-FLAG in nf-yc9-1 pNF-YC9:NF-YC9-FLAG ( Fig. 4c ). However, ChIP assays of nf-yc9-1 pNF-YC9:NF-YC9-FLAG revealed that NF-YC9-FLAG binding to the SOC1 promoter was significantly enhanced or compromised by GA or PAC treatment, respectively ( Fig. 4d ). Thus, GA signalling regulates flowering through enhancing NF-Y binding to SOC1 rather than affecting the expression levels of NF-Y proteins. NF-Y reduces H3K27me3 levels at SOC1 Although several studies have correlated NF-Y binding to histone marks at downstream genes [41] , [42] , [43] , it is so far unclear whether NF-Y affects histone modifications in plants. To understand how NF-Y regulates SOC1 transcription, we compared the distribution profiles of several selected histone marks, including H3ac, H4ac, H3K4me2, H3K4me3, H3K9ac and H3K27me3, at the SOC1 locus between wild-type and nf-ya2-1 nf-yb2-1 nf-yb3-1 nf-yc9-1 plants by ChIP assays. While these histone marks were all enriched to different extents at SOC1 , H3K27me3 exhibited the most dramatic change in its levels in nf-ya2-1 nf-yb2-1 nf-yb3-1 nf-yc9-1 as compared with wild-type plants ( Fig. 5a , Supplementary Fig. 14 ). H3K27me3 is a histone mark associated with transcriptionally silent chromatin, which is specifically recognized by TERMINAL FLOWER 2 (TFL2), the only Arabidopsis homologue of HP1 (ref. 44 ). ChIP analysis using tfl2-1 35S:TFL2-3HA [45] showed the association of TFL2-3HA with SOC1 at the same region ( SOC1-10 ) highly enriched for H3K27me3 ( Fig. 5a,b ), confirming the deposition of H3K27me3 at SOC1 . The progressive increase of H3K27me3 levels at SOC1 in nf-yb2-1 nf-yb3-1 and nf-ya2-1 nf-yb2-1 nf-yb3-1 nf-yc9-1 ( Fig. 5a ) was consistent with decreased expression of SOC1 in these mutants ( Fig. 2a ), suggesting that NF-Y subunits might play a redundant role in affecting H3K27me3 levels at SOC1 . In addition, H3K27me3 levels also greatly increased at SOC1 in co-1 and ga1 ( Fig. 5c ). These results indicate that the effect of CO and GA signalling on SOC1 mediated by NF-Y is associated with H3K27me3 levels at SOC1 . 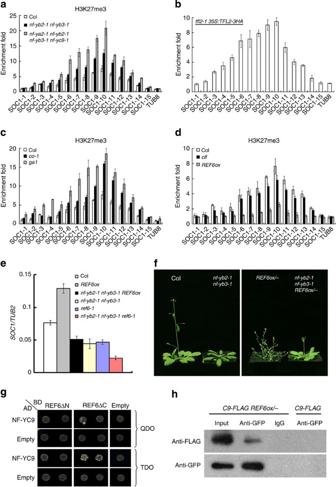Figure 5: NF-Y affects H3K27me3 dynamics atSOC1and interacts with REF6. (a) NF-Y affects H3K27me3 levels atSOC1. ChIP analysis of H3K27me3 levels was performed with 9-day-old plants grown under LDs. Values are mean±s.d. of three biological replicates. (b) ChIP analysis of TFL2-3HA binding to theSOC1regulatory regions. Nine-day-oldtfl2-1 35S:TFL2-3HAplants were collected for ChIP analysis. (c,d) ChIP analysis of H3K27me3 levels atSOC1inco-1andga1(c), or inclfandREF6-YFP-HAoverexpression plants (REF6ox) (d). Nine-day-old plants were collected for ChIP analysis. (e) Quantitative RT–PCR analysis ofSOC1expression in 9-day-old plants with various genetic backgrounds under LDs.TUB2was amplified as an internal control. Values are mean±s.d. of three biological replicates. (f)nf-yb2-1 nf-yb3-1partially suppresses early flowering ofREF6ox. Flowering phenotypes of representative 29-day-old plants with various genetic backgrounds grown under LDs were compared. AsREF6oxhomozygous plants are very tiny and flower extremely early, the phenotypic comparison was made among plants with theREF6oxheterozygous background (REF6ox/−). (g) Yeast two-hybrid assays show the interaction between NF-YC9 and the N terminus of REF6. Transformed yeast cells were grown on SD-Trp/-Leu/-His (TDO) or SD-Trp/-Leu/-His/-Ade medium (QDO). (h)In vivointeraction between NF-YC9 and REF6 inArabidopsis. Plant nuclear extracts from 9-day-oldnf-yc9-1 pNF-YC9:NF-YC9-FLAGandnf-yc9-1 pNF-YC9:NF-YC9-FLAG REF6ox/−seedlings were immunoprecipitated by anti-GFP antibody or preimmune serum (IgG). The co-immunoprecipitated proteins were detected by anti-FLAG or anti-GFP antibody as indicated on the left of each blot.C9-FLAG,nf-yc9-1 pNF-YC9:NF-YC9-FLAG. Figure 5: NF-Y affects H3K27me3 dynamics at SOC1 and interacts with REF6. ( a ) NF-Y affects H3K27me3 levels at SOC1 . ChIP analysis of H3K27me3 levels was performed with 9-day-old plants grown under LDs. Values are mean±s.d. of three biological replicates. ( b ) ChIP analysis of TFL2-3HA binding to the SOC1 regulatory regions. Nine-day-old tfl2-1 35S:TFL2-3HA plants were collected for ChIP analysis. ( c , d ) ChIP analysis of H3K27me3 levels at SOC1 in co-1 and ga1 ( c ), or in clf and REF6-YFP-HA overexpression plants ( REF6ox ) ( d ). Nine-day-old plants were collected for ChIP analysis. ( e ) Quantitative RT–PCR analysis of SOC1 expression in 9-day-old plants with various genetic backgrounds under LDs. TUB2 was amplified as an internal control. Values are mean±s.d. of three biological replicates. ( f ) nf-yb2-1 nf-yb3-1 partially suppresses early flowering of REF6ox . Flowering phenotypes of representative 29-day-old plants with various genetic backgrounds grown under LDs were compared. As REF6ox homozygous plants are very tiny and flower extremely early, the phenotypic comparison was made among plants with the REF6ox heterozygous background ( REF6ox/−) . ( g ) Yeast two-hybrid assays show the interaction between NF-YC9 and the N terminus of REF6. Transformed yeast cells were grown on SD-Trp/-Leu/-His (TDO) or SD-Trp/-Leu/-His/-Ade medium (QDO). ( h ) In vivo interaction between NF-YC9 and REF6 in Arabidopsis . Plant nuclear extracts from 9-day-old nf-yc9-1 pNF-YC9:NF-YC9-FLAG and nf-yc9-1 pNF-YC9:NF-YC9-FLAG REF6ox/− seedlings were immunoprecipitated by anti-GFP antibody or preimmune serum (IgG). The co-immunoprecipitated proteins were detected by anti-FLAG or anti-GFP antibody as indicated on the left of each blot. C9-FLAG , nf-yc9-1 pNF-YC9:NF-YC9-FLAG . Full size image To further examine the relationship between NF-Y and the H3K27me3 status at SOC1 , we measured H3K27me3 levels at the native and mutated pSOC1:GUS transgene loci in the native and mutated pSOC1:GUS plants, respectively ( Fig. 3d ). H3K27me3 levels were much higher at the mutated locus ( Supplementary Fig. 15 ), indicating that NFYBE bound by NF-Y is involved in mediating H3K27me3 levels at SOC1 . NF-Y mediates H3K27me3 demethylation at SOC1 partly via REF6 Because H3K27me3 is deposited by H3K27me3 methyltransferases of the polycomb repressive complex 2 and removed by H3K27 demethylases, we then examined whether NF-Y modulates H3K27me3 dynamics at SOC1 through its interaction with CURLY LEAF (CLF), a main H3K27me3 methyltransferase, or REF6, a H3K27 demethylase, both of which affect flowering in Arabidopsis ( Table 1 ) [46] , [47] , [48] , [49] . As both clf and REF6-YFP-HA overexpression ( REF6ox ) plants exhibit global changes in H3K27me3 levels [46] , [47] , we performed ChIP assays on these two types of plants and found that overexpression of REF6 dramatically reduced H3K27me3 levels at SOC1 , whereas there was no significant change in H3K27me3 levels in clf ( Fig. 5d ). Although REF6 was also reported to act as an H3K4me3/H3K36me3 demethylase [50] , we did not observe significant changes in H3K4me3/H3K36me3 levels at SOC1 in both REF6ox and ref6-1 compared with wild-type plants ( Supplementary Fig. 16 ). In agreement with REF6 role in reducing H3K27me3 levels, SOC1 was upregulated in REF6ox and slightly downregulated in ref6-1 ( Fig. 5e ). In contrast, SOC1 was unexpectedly downregulated in clf ( Supplementary Fig. 17 ), which could indirectly result from the effect of CLF on SOC1 upstream regulators, such as FLOWERING LOCUS C [46] . Having shown that both NF-Y and REF6 promoted SOC1 expression through reducing H3K27me3 levels ( Fig. 5a,d,e ), we crossed nf-yb2-1 nf-yb3-1 with REF6ox and ref6-1 to investigate whether NF-Y interacts with REF6 to affect SOC1 expression. Upregulation of SOC1 in REF6ox was attenuated by nf-yb2-1 nf-yb3-1 ( Fig. 5e ), which is consistent with the observation that nf-yb2-1 nf-yb3-1 partially suppressed the extremely early flowering phenotype of REF6ox ( Fig. 5f , Table 1 ). Furthermore, SOC1 expression was lower in nf-yb2-1 nf-yb3-1 ref6-1 than in nf-yb2-1 nf-yb3-1 and ref6-1 ( Fig. 5e ). Consequently, the late-flowering phenotype of ref6-1 was enhanced by nf-yb2-1 nf-yb3-1 ( Table 1 ). These results support that NF-Y partially mediates REF6 effect on SOC1 expression. As NF-Y did not affect mRNA expression of REF6 ( Supplementary Fig. 18 ), we then tested the protein interaction between a NF-Y subunit, NF-YC9 and REF6. Yeast two-hybrid assay revealed the interaction between NF-YC9 and the amino terminus of REF6 in yeast ( Fig. 5g ), and co-immunoprecipitation analysis of nf-yc9-1 pNF-YC9:NF-YC9-FLAG REF6ox/− plants confirmed the interaction between NF-YC9 and REF6 in Arabidopsis ( Fig. 5h ). These findings suggest that NF-Y interacts with REF6 to regulate SOC1 expression. Consistently, reduction of H3K27me3 levels at SOC1 in REF6ox was suppressed by nf-yb2-1 nf-yb3-1 , while H3K27me3 levels significantly increased in nf-yb2-1 nf-yb3-1 ref6-1 compared with those in ref6-1 and nf-yb2-1 nf-yb3-1 ( Fig. 6a ). 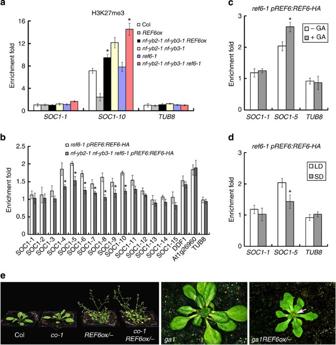Figure 6: Interaction between REF6 and NF-Y directly regulatesSOC1expression downstream of photoperiod and GA pathways. (a) ChIP analysis of H3K27me3 levels atSOC1in various genetic backgrounds. Nine-day-old plants grown under LDs were collected for ChIP analysis. Values are mean±s.d. of three biological replicates. Asterisks indicate significant changes in ChIP-enrichment fold innf-yb2-1 nf-yb3-1 REF6oxcompared withREF6ox, or innf-yb2-1 nf-yb3-1 ref6-1compared withnf-yb2-1 nf-yb3-1andref6-1(two-tailed Student’st-test,P<0.05). (b) ChIP analysis of REF6-HA binding to theSOC1regulatory regions. Nine-day-oldref6-1 pREF6:REF6-HAandnf-yb2-1 nf-yb3-1 ref6-1 pREF6:REF6-HAgrown under LDs were collected for ChIP analysis.nf-yb2-1nf-yb3-1 ref6-1 pREF6:REF6-HAwas generated from a cross betweennf-yb2-1 nf-yb3-1andref6-1 pREF6:REF6-HA, and exhibited comparable flowering time tonf-yb2-1 nf-yb3-1(Table 1). Two known targets,DDF1andAt1g26960, bound by REF6-6HA47served as positive controls in ChIP assays. Values are mean±s.d. of three biological replicates. Asterisks indicate significant changes in ChIP-enrichment fold innf-yb2-1 nf-yb3-1 ref6-1 pREF6:REF6-HAcompared withref6-1 pREF6:REF6-HA(two-tailed Student’st-test,P<0.05). In agreement with NF-Y binding profile (Fig. 3a), REF6-HA is associated withSOC1-5with the highest enrichment fold. (c,d) ChIP analysis of REF6-HA binding to theSOC1regulatory regions in response to GA (c) and photoperiod (d). Nine-day-oldref6-1 pREF6:REF6-HAplants grown under LDs treated with 100 μM GA3for 24 h (c) or grown under short days (SDs) (d) were collected for ChIP analysis. Nine-day-oldref6-1 pREF6:REF6-HAgrown under LDs without GA treatment served as a control for both ChIP analyses shown in (c,d). Values are mean±s.d. of three biological replicates. Asterisks indicate significant changes in ChIP-enrichment fold in comparison with respective controls (two-tailed Student’st-test,P<0.05). (e)REF6oxsuppresses late flowering ofco-1andga1. The left panel shows representative 27-day-old Col,co-1,REF6ox/−andco-1 REF6ox/−plants, while the middle and right panels show a 29-day-oldga1mutant and a 22-day-oldga1 REF6ox/−plant, respectively. Arrow indicates floral buds inga1 REF6ox/−. Figure 6: Interaction between REF6 and NF-Y directly regulates SOC1 expression downstream of photoperiod and GA pathways. ( a ) ChIP analysis of H3K27me3 levels at SOC1 in various genetic backgrounds. Nine-day-old plants grown under LDs were collected for ChIP analysis. Values are mean±s.d. of three biological replicates. Asterisks indicate significant changes in ChIP-enrichment fold in nf-yb2-1 nf-yb3-1 REF6ox compared with REF6ox , or in nf-yb2-1 nf-yb3-1 ref6-1 compared with nf-yb2-1 nf-yb3-1 and ref6-1 (two-tailed Student’s t -test, P <0.05). ( b ) ChIP analysis of REF6-HA binding to the SOC1 regulatory regions. Nine-day-old ref6-1 pREF6:REF6-HA and nf-yb2-1 nf-yb3-1 ref6-1 pREF6:REF6-HA grown under LDs were collected for ChIP analysis. nf-yb2-1nf-yb3-1 ref6-1 pREF6:REF6-HA was generated from a cross between nf-yb2-1 nf-yb3-1 and ref6-1 pREF6:REF6-HA , and exhibited comparable flowering time to nf-yb2-1 nf-yb3-1 ( Table 1 ). Two known targets, DDF1 and At1g26960 , bound by REF6-6HA [47] served as positive controls in ChIP assays. Values are mean±s.d. of three biological replicates. Asterisks indicate significant changes in ChIP-enrichment fold in nf-yb2-1 nf-yb3-1 ref6-1 pREF6:REF6-HA compared with ref6-1 pREF6:REF6-HA (two-tailed Student’s t -test, P <0.05). In agreement with NF-Y binding profile ( Fig. 3a ), REF6-HA is associated with SOC1-5 with the highest enrichment fold. ( c , d ) ChIP analysis of REF6-HA binding to the SOC1 regulatory regions in response to GA ( c ) and photoperiod ( d ). Nine-day-old ref6-1 pREF6:REF6-HA plants grown under LDs treated with 100 μM GA 3 for 24 h ( c ) or grown under short days (SDs) ( d ) were collected for ChIP analysis. Nine-day-old ref6-1 pREF6:REF6-HA grown under LDs without GA treatment served as a control for both ChIP analyses shown in ( c , d ). Values are mean±s.d. of three biological replicates. Asterisks indicate significant changes in ChIP-enrichment fold in comparison with respective controls (two-tailed Student’s t -test, P <0.05). ( e ) REF6ox suppresses late flowering of co-1 and ga1 . The left panel shows representative 27-day-old Col, co-1 , REF6ox/− and co-1 REF6ox/− plants, while the middle and right panels show a 29-day-old ga1 mutant and a 22-day-old ga1 REF6ox/− plant, respectively. Arrow indicates floral buds in ga1 REF6ox/− . Full size image ChIP assays using a previously established ref6-1 pREF6:REF6-HA transgenic line, in which a functional version of REF6-HA rescued the flowering defect of ref6-1 (ref. 47 ) showed that REF6-6HA was associated with SOC1 , and that this association was significantly attenuated in nf-yb2-1 nf-yb3-1 and under SD conditions ( Fig. 6b,d ), but enhanced by GA treatment ( Fig. 6c ). These data, together with the observation that overexpression of REF6 dramatically suppressed late flowering of co-1 and ga1 ( Fig. 6e , Table 1 ), substantiate that the interaction between REF6 and NF-Y directly regulates SOC1 downstream of CO and GA signalling. Combinatorial transcription factors, such as NF-Y complexes, play an essential role in regulating eukaryotic gene expression [51] . Unlike other eukaryotic organisms, the plant lineage has multiple genes that encode each subunit of a heterotrimeric NF-Y complex [32] , [34] . Individual plant NF-Y subunits have been shown to affect various developmental processes and plant responses to environmental stresses [28] , [29] , [30] , [52] , [53] , [54] , [55] . However, the precise function of complete NF-Y complexes in plants so far remains elusive. Here we show a NF-Y complex composed of three different types of subunits, NF-YA2, NF-YB2 and NF-YC9, which controls flowering time through directly regulating SOC1 transcription in response to flowering signals from photoperiod and GA pathways in Arabidopsis ( Fig. 7 ). nf-ya2-1 nf-yb2-1 nf-yb3-1 nf-yc9-1 exhibits much later flowering than nf-yb2-1 nf-yb3-1 ( Table 1 ), indicating that these NF-Y subunits play redundant roles in promoting flowering. NF-YB and NF-YC subunits interact with CO in the photoperiod pathway as previously reported [28] , [29] , and also with RGA in the GA pathway. Among the NF-Y subunits examined, NF-YC9 serves as a key component that not only mediates the interaction between NF-YA2 and NF-YB2 in the NF-Y heterotrimer ( Fig. 1d ), but also interacts in vivo with CO and RGA ( Fig. 1e ). A recent study has suggested that plant NF-YC enables translocation of NF-YB to the nucleus, and that the resulting NF-YB/NF-YC heterodimer is required for further recruitment of NF-YA in the final assembly of the heterotrimeric NF-Y complex as shown in mammals [35] . Thus, our finding of NF-YC9 as a common partner of other NF-Y subunits, CO, and RGA implies that NF-YC9 could be a key subunit that coordinates the perception of flowering signals and the assembly of the specific combinatorial NF-Y transcription factor that triggers the downstream regulatory events in response to flowering signals. 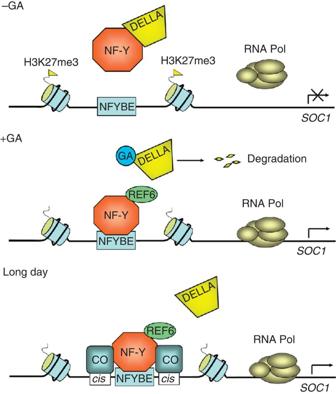Figure 7: Photoperiod and GA pathways regulateSOC1expression via NF-Y-mediated H3K27me3 demethylation. Without GA, stabilized DELLAs interact with the NF-Y complex and inhibit NF-Y binding to the NFYBE at theSOC1locus. This compromises NF-Y-dependent demethylation of H3K27me3, thus repressingSOC1expression. Degradation of DELLAs triggered by GA liberates NF-Y to bind to the NFYBE. NF-Y then recruits REF6 to demethylate H3K27me3 atSOC1, thus promotingSOC1expression. Under LD conditions, stabilized CO protein interacts with NF-Y regardless of the presence of DELLAs. Both of CO and NF-Y bind to theSOC1regulatory regions, which facilitates NF-Y-mediated demethylation of H3K27me3 and promotesSOC1expression. Figure 7: Photoperiod and GA pathways regulate SOC1 expression via NF-Y-mediated H3K27me3 demethylation. Without GA, stabilized DELLAs interact with the NF-Y complex and inhibit NF-Y binding to the NFYBE at the SOC1 locus. This compromises NF-Y-dependent demethylation of H3K27me3, thus repressing SOC1 expression. Degradation of DELLAs triggered by GA liberates NF-Y to bind to the NFYBE. NF-Y then recruits REF6 to demethylate H3K27me3 at SOC1 , thus promoting SOC1 expression. Under LD conditions, stabilized CO protein interacts with NF-Y regardless of the presence of DELLAs. Both of CO and NF-Y bind to the SOC1 regulatory regions, which facilitates NF-Y-mediated demethylation of H3K27me3 and promotes SOC1 expression. Full size image Our results suggest that the CO-mediated photoperiod pathway and GA signalling function in parallel in promoting flowering under LDs. The integration of plant responses to these two pathways converges on the NF-Y complex. The genetic data showing the similar late-flowering phenotype of nf-yb2-1 nf-yb3-1 and nf-yb2-1 nf-yb3-1 co-1 and complete suppression of early flowering of SUC2:CO-6HA by nf-yb2-1 nf-yb3-1 suggest that CO regulates flowering in a NF-Y-dependent manner. Consistent with the protein interaction between NF-Y and CO, the SOC1 promoter region associated with NF-Y subunits overlaps with the region bound by CO. Furthermore, the NFYBE in the SOC1 promoter bound by NF-Y is required for the upregulation of SOC1 by CO. These observations all support that NF-Y is an important regulator that mediates CO effect on SOC1 transcription ( Fig. 7 ). In contrast to CO, RGA in the GA pathway represses SOC1 transcription. Although RGA interacts with NF-Y, RGA does not directly bind to the SOC1 promoter. GA treatment degrades RGA, which enhances NF-Y binding to SOC1 . These results suggest that DELLA proteins, such as RGA, affect SOC1 expression through preventing NF-Y binding to SOC1 ( Fig. 7 ). This is substantiated by the observations that the NFYBE in the SOC1 promoter is indispensable for upregulation of SOC1 by GA treatment ( Fig. 3d,e ), and that the flowering response to GA is partially compromised in nf-ya2-1 nf-yb2-1 nf-yb3-1 nf-yc9-1 ( Supplementary Table 1 ). In addition to SOC1 , the GA pathway also affects other components of the regulatory network that integrates flowering signals. For example, GA plays spatially distinct regulatory roles in promoting transcription of FT and SPL genes under LDs [21] , [56] . It has been demonstrated that NF-Y complexes bind to the CCAAT box, a cis-element present in nearly 25% of eukaryotic promoters, indicating that NF-Y complexes are involved in transcriptional regulation of a considerable number of eukaryotic genes [33] , [42] , [57] . Several studies have tested in vitro binding sites of plant NF-Y subunits [55] , [58] , but whether these sites are relevant to NF-Y endogenous function is unclear. Another recent study has proposed that NF-Y complexes may recognize a distal CCAAT site at the FT promoter based on ChIP assays of 35S:NF-YB2-YFP/HA plants [59] , whereas we were unable to detect binding of NF-YB2-6Myc to FT using the nf-yb2-1 pNF-YB2:NF-YB2-6Myc tagging line ( Supplementary Fig. 9 ). We show here that the NF-YA2/NF-YB2/NF-YC9 complex binds to a unique NFYBE, 5′-TTCACAAACACCATT-3′, through NF-YA2. It is noteworthy that this NFYBE does not contain the exact NF-Y consensus binding site, CCAAT, as shown in yeast and animals, implying that the diversity in plant NF-Y subunits may evolve with the divergence of their corresponding cis -elements. The SOC1 genomic region containing the NFYBE demonstrates two unique features that are relevant to regulation of SOC1 by CO and GA signalling. First, it has been proposed that CO activates SOC1 through being recruited by a DNA-binding factor to a motif located between nt −372 and −248 in the SOC1 promoter [18] . This region exactly overlaps with the SOC1-5 fragment containing the newly identified NFYBE, implying that NF-Y could be the long-sought DNA-binding factor for CO. Furthermore, CO has been shown to bind a CO-responsive element containing a consensus TGTG(N2-3)ATG motif in the FT promoter [60] . Notably, there are two similar motifs (TGTGTATG) located 199 bp upstream and 262 bp downstream from the NFYBE in the SOC1 promoter, respectively. The entire region containing these motifs is associated with CO in vivo ( Fig. 3a ). In concert, these results suggest that CO and NF-Y interact at the same region centred on the NFYBE to activate SOC1 transcription. Second, the forepart of the NFYBE is similar to a GA-responsive cis -element (GARE), 5′-TAACAAA/G-3′, which has been identified from an α-amylase gene in barley aleurone layers [61] . This element is bound by GAMYB, a GA-inducible transcriptional factor, which activates the α-amylase gene expression in aleurone cells [62] . In Arabidopsis , the GARE is significantly enriched in the promoters of GA-responsive genes [63] . AtMYB33, a GAMYB protein, has been suggested to promote flowering through binding to a GARE-like element in the LFY promoter [64] . Thus, it is tempting to speculate that the interaction between DELLAs and NF-Y may also affect NF-Y interaction with other GARE-binding trans -acting partners at the NFYBE, thus mediating the downstream response of GA signalling in plants. NF-YB and NF-YC subunits have conserved histone fold motifs that resemble H2B and H2A, respectively, both of which, together with H3 and H4, are core histones of the nucleosome, the fundamental unit of chromatin [65] . In yeast and animals, NF-Y could modulate chromatin structure and function through replacement of H2A-H2B and/or covalent modifications of histones, such as methylation and acetylation [33] . One of the most intriguing questions relevant to NF-Y function is how the interaction between NF-Y and other transcriptional regulators mediates spatial and temporal regulation of selected specific loci rather than bulk chromatin. In this study, we show that a plant NF-Y complex plays an important role in integrating environmental and developmental signals to govern the selection of a specific key regulator to be targeted by a general histone demethylase. NF-Y mediates the effect of photoperiod and GA signalling on SOC1 expression partly through modulating H3K27me3 demethylation via a H3K27 demethylase REF6. Both CO and RGA interact with NF-Y that directly binds to the NFYBE in the SOC1 promoter, which in turn mediates REF6 to modulate H3K27me3 levels at SOC1 . Our findings establish NF-Y as a key complex that orchestrates plant responses to seasonal changes in day length and the endogenous phytohormone GA to mediate epigenetic control of the floral transition in a locus-specific manner. As different combinations of multiple NF-Y subunits may result in the formation of various NF-Y complexes with different intrinsic properties and trans -acting partners, this flexibility could allow plants to respond and adapt to various stresses through controlling a large number of specific targets at the molecular level, although they cannot move away from stressful environments. Plant materials and growth conditions Arabidopsis plants were grown at 22 °C under LDs (16 h light/8 h dark) or short days (8 h light/16 h dark). The mutants ga1-3 , rga-t2 , gai-t6 , rgl1-1 , rgl2-1 and co-2 are in L er background, while all the other mutants are in Col background. nf-yb2-1 (SALK_025666), nf-yb3-1 (SALK_062245), nf-yc9-1 (SALK_058903), nf-yc4-1 (SALK_032163) and clf (SALK_006658) seeds were obtained from the Arabidopsis Biological Resource Centre, while nf-ya2-1 (GK-440G05) and nf-yc3-2 (GK-051E10) were obtained from the European Arabidopsis Stock Centre. Seeds with ga1-3 or ga1 background were imbibed in 100 μM GA 3 at 4 °C for 7 days and rinsed thoroughly with water before sowing. Plasmid construction and plant transformation To construct 35S:NF-YC9-6HA , 35S:NF-YC3-6HA and 35S:NF-YA2-6HA , the cDNAs encoding NF-YC9, NF-YC3 and NF-YA2 were amplified and cloned into pGreen-35S-6HA, respectively [5] . To construct pNF-YC9: NF-YC9-FLAG and pNF-YB2:NF-YB2-6Myc , the genomic fragments of NF-YC9 and NF-YB2 were amplified and cloned into pHY105-6Myc and pPZPY122-FLAG [26] , respectively. The SUC2 promoter fragment and the cDNA encoding CO were amplified and cloned into pHY105-6HA to obtain SUC2:CO-6HA . For the complementation test, a 6.6-kb SOC1 genomic fragment that includes 2.4 kb of the upstream sequence, 3.5 kb of the transcribed region, and 0.7 kb of the 3′-flanking region was amplified and cloned into pHY105 (ref. 5 ) to obtain the gSOC1 construct. Based on the native gSOC1 and the previously reported pSOC1:GUS constructs [5] , the derived constructs with the mutated NFYBE were produced using QuikChange II XL-Site-Directed Mutagenesis Kit (Stratagene). Primers used for plasmid construction are listed in Supplementary Table 2 . Except for transgenic plants harbouring pNF-YC9:NF-YC9-FLAG that were selected on MS medium supplemented with gentamicin, transgenic plants with other constructs were selected by Basta on soil. Yeast two-hybrid and three-hybrid assays The coding regions of NF-YC1 , NF-YC9, NF-YC3 , NF-YB1 , NF-YB2, NF-YB3, NF-YA1, NF-YA2, CO and DELLAs were amplified and cloned into either pGBKT7 or pGADT7 (Clontech). Yeast two-hybrid assays were performed using the Yeastmaker Yeast Transformation System 2 (Clontech). To screen an Arabidopsis cDNA library (CD4-30, from ABRC) [66] , the fragment of RGAΔN (residues 200–587) was fused to the GAL4-BD as bait. To analyse the interaction between NF-YC9 and REF6, the carboxy- and N-terminal fragments of REF6 were amplified and cloned into pGBKT7 to obtain BD-REF6ΔN and BD-REF6ΔC , respectively. To analyse the formation of the trimeric NF-Y complex, the NF-YC9 coding region was amplified and cloned into pQH05, which was derived from pTH184 with a HIS3 selection marker. Primers used for generating constructs for yeast two-hybrid and three-hybrid assays are listed in Supplementary Table 2 . Yeast AH109 cells were co-transformed with specific bait and prey constructs. For yeast three-hybrid assay, yeast AH109 cells were co-transformed with AD-NF-YB2/NF-YB3 and BD-NF-YA1/NF-YA2 in the presence of either pQH05 or pQH05-NF-YC9. All yeast transformants were grown on SD/-Trp/-Leu/-His/-Ade medium for selection or interaction test. Expression analysis Total RNA was extracted using the FavorPre Plant Total RNA Mini Kit (Favorgen) and reverse transcribed using the SuperScrip RT–PCR System (Invitrogen). Real-time PCR was performed in triplicates on CFX38 real-time system (Bio-Rad) with the iQ SYBR Green Supermix (Bio-Rad). The relative expression level was calculated as previously reported [5] . Primers used for gene expression analysis are listed in Supplementary Table 2 . GUS staining and quantitative analysis of GUS activity were carried out as previously described [67] . In vitro pull-down assay To produce GST-tagged proteins, the cDNAs encoding RGA and CO were cloned into pGEX-4T-1 vector (Pharmacia). To produce His-tagged proteins, the cDNAs encoding NF-YC9, NF-YB2 and NF-YA2 were cloned into pQE30 vector (Qiagen). Primers used for these constructs are listed in Supplementary Table 2 . These constructs and the empty pGEX-4T-1 and pQE30 vectors were transformed into E. coli Rosetta (DE3) (Novagen), and protein expression was induced by IPTG. The soluble His fusion proteins were immobilized onto Ni-NTA agarose beads (30210, Qiagen), while the soluble GST fusion proteins were immobilized onto glutathione sepharose beads (17-0756-01, Amersham Biosciences). For pull-down assays, 2 μg His fusion proteins were incubated with the immobilized GST and GST fusion proteins at 4 °C for 1 h. Proteins retained on the beads were subsequently resolved by SDS–polyacrylamide gel electrophoresis and detected with anti-His antibody (Santa Cruz Biotechnology). Uncropped scans of western blot results are shown in Supplementary Fig. 19 . ChIP assay Nine-day-old seedlings with various genetic backgrounds were fixed on ice for 45 min in 1% formaldehyde under vacuum. Fixed tissues were homogenized, and chromatin was isolated and sonicated as previously described [5] . The solubilized chromatin was immunoprecipitated by either a specific antibody or mouse IgG (15,381, Sigma) with Protein G PLUS agarose (sc-2002, Santa Cruz Biotechnology). NF-YC9-FLAG, NF-YB2-6Myc, NF-YA2-6HA and CO-6HA were immunoprecipitated by anti-FLAG (A2220, Sigma), anti-Myc (A7470, Sigma) and anti-HA agarose conjugates (A2095, Sigma), respectively. Various histone modifications were detected by anti-H3K27me3 (07-449, Millipore), anti-H3K4me2 (07-030, Millipore), anti-H3K4me3 (07-473, Millipore), anti-H3K36me3 (ab9050, Abcam), anti-H3K9ac (06-942, Millipore), anti-Acetyl-H3 (06-599, Millipore) and anti-Acetyl-H4 antibodies (06-866, Millipore). The co-immunoprecipitated DNA was recovered and analysed by quantitative real-time PCR in triplicates. For ChIP assays of H3K27me3 levels and binding of CO and various NF-Y subunits to SOC1 , relative fold enrichment was calculated by normalizing the amount of a target DNA fragment against that of a genomic fragment of a reference gene, ACTIN7 ( At5g09810 ), and then by normalizing the value for immunoprecipitation using a specific antibody against that of mouse IgG. The enrichment of a Tubulin ( TUB8 ; At5g23860 ) genomic fragment was used as a negative control. For ChIP assays of H3ac, H4ac, H3K4me2, H3K4me3, H3K36me3 and H3K9ac levels, Ta2 transposon ( At4g06488 ) served as a reference gene, while the enrichment of a Cinful-like ( At4g03770 ) genomic fragment was used as a negative control [68] . Co-immunoprecipitation assay Nine-day-old seedlings with various genetic backgrounds were collected, and nuclear proteins were extracted according to the ChIP protocol but without the tissue fixation step. NF-YC9-FLAG was immunoprecipitated by anti-FLAG agarose conjugate (A2220, Sigma), anti-Myc agarose conjugate (A7470, Sigma), or anti-GFP antibody (A11122, Invitrogen). Proteins bound to the beads were resolved by SDS–polyacrylamide gel electrophoresis and detected by anti-Myc (SAB4700447, Sigma), anti-FLAG (F3165, Sigma), anti-HA (H9658, Sigma), or anti-GFP antibody (A11122, Invitrogen). Uncropped scans of Western blot results are shown in Supplementary Fig. 19 . BiFC analysis The cDNAs of the proteins tested were cloned into serial pSAT1 vectors containing either N- or C-terminal-enhanced yellow fluorescence protein fragments. The resulting cassettes were further subcloned into a pGreen binary vector HY105 for BiFC analysis as previously published [61] . EMSA EMSA assay was performed using the LightShift Chemiluminescent EMSA kit (Pierce). The SOC1-5 fragment or the double-stranded oligonucleotides of the native and mutated NF-YA2 binding element in the SOC1 promoter with 13 bp flanking sequences at both ends [69] were biotin end labelled and used as probes. Non-labelled probes were used as cold competitors. How to cite this article : Hou, X. et al. Nuclear factor Y-mediated H3K27me3 demethylation of the SOC1 locus orchestrates flowering responses of Arabidopsis . Nat. Commun. 5:4601 doi: 10.1038/ncomms5601 (2014).